Solvent-triggered reversible interconversion of all-nitrogen-donor-protected silver nanoclusters and their responsive optical properties Surface organic ligands are critical in determining the formation and properties of atomically precise metal nanoclusters. In contrast to the conventionally used thiolate, phosphine and alkynyl ligands, the amine ligand dipyridylamine is applied here as a protecting agent in the synthesis of atomically precise metal nanoclusters. We report two homoleptic amido-protected Ag nanoclusters as examples of all-nitrogen-donor-protected metal nanoclusters: [Ag 21 (dpa) 12 ]SbF 6 ( Ag 21 ) and [Ag 22 (dpa) 12 ](SbF 6 ) 2 ( Ag 22 ) (dpa = dipyridylamido). Single crystal X-ray structural analysis reveals that both clusters consist of a centered-icosahedron Ag 13 core wrapped by 12 dpa ligands. The flexible arrangement of the N donors in dpa facilitates the solvent-triggered reversible interconversion between Ag 21 and Ag 22 due to their very different solubility. The successful use of dpa in the synthesis of well-defined silver nanoclusters may motivate more studies on metal nanoclusters protected by amido type ligands. Along with the advance of synthetic methodologies of ligand passivated nanoparticles in the past decades [1] , intense attention is also paid to synthesize atomically precise nanoclusters. The precise control over number of atoms and their arrangements within the clusters could provide valuable possibilities in modulating the various properties of nanoclusters [2] , [3] , [4] , [5] , [6] , [7] , [8] , [9] , [10] . The isolation of metal nanoclusters needs the protection from organic/inorganic, which play important roles in determining the stability, atom packing, and properties of metal clusters. Phosphine [11] , [12] , [13] , [14] , [15] , thiolate [16] , [17] , [18] , [19] , [20] , [21] , [22] , [23] , and alkynyl ligands [24] , [25] , [26] , [27] , [28] , [29] , [30] have been extensively used in the synthesis of metal nanoclusters, but the detailed amido-metal interfaces are still elusive due to the lack of total structural determination of amido-protected metal nanoclusters [31] , [32] , [33] . The unveiling of metal-amine interface will not only be helpful for understanding the formation of related clusters and establishing structure-property relationships, but also provides valuable information for the controlled synthesis of nanoparticles. In order to isolate a stable amido-protected metal nanocluster, which is helpful for making structural determination possible, our strategy is to use dipyridylamine (Hdpa) as a multidentate protecting agent. After deprotonation, Hdpa turns into a monoanionic dipyridylamido (dpa) ligand, which contains one amido and two pyridyl N donors available for bridging multi metal centers. The two pyridyl groups provide additional binding sites for metal atoms, which is advantageous in stabilizing metal clusters. On the other hand, many factors have been found influencing the formation of metal clusters, such as ligand hindrance, temperature and pH values. Ligand hindrance has been demonstrated to control the size of Au n (SR) m nanoclusters [34] . Au 130 ( p -MBT) 50 , Au 104 ( m -MBT) 41 , and Au 40 ( o -MBT) 24 nanoclusters were obtained with methylbenzenethiols (MBT) as a result of their different positions of the methyl groups. A metastable Au 38 (SC 2 H 4 Ph) 24 isolated at low temperature could be irreversibly converted to biicosahedral isomer at 50 °C [19] . Captopril (Capt) ligand stabilized Au 25 Capt 18 was transformed into highly fluorescent Au 23 Capt 17 under treatment of HCl [35] . Solvents were also demonstrated to be important in some cases, e.g. an icosahedral-to-cuboctahedral structural transition was achieved by adding hexane into an ethanol solution of Au 13 (PPh 3 ) 4 (SC 12 H 25 ) 4 (SC 12 H 25 = dodecanethiol) [36] . Herein, we report an interesting case that reversible interconversion of clusters can be triggered by different solvents. With the protection of dpa, we are able to isolate all-amido-protected Ag nanoclusters: [Ag 21 (dpa) 12 ]SbF 6 ( Ag 21 ) and [Ag 22 (dpa) 12 ](SbF 6 ) 2 ( Ag 22 ). The total structural determination of the clusters have been carried out. To our surprise, it is found that Ag 21 and Ag 22 can be reversibly interconverted via solvent triggers, i.e., the transformation may be induced by solvents, due to their different solubility. Both clusters have very similar structures based on a centered-icosahedral Ag 13 core, with different number of shell silver atoms ligated by the same number of homoleptic dpa ligands. Although Ag 21 and Ag 22 have similar structures, they display significantly different optical properties. Synthesis The preparation of Ag 21 involves the reduction of the dpa-Ag precursor in the presence of phosphine, Hdpa, AgSbF 6 , and MeONa in dichloromethane. Similarly, the Ag 22 cluster can be obtained without addition of Hdpa, and the amount of NaBH 4 should be decreased (see Supporting Information). Although phosphines did not appear in the resulted clusters, they are important for the preparation. We monitored the 31 P spectra in the synthesis of Ag 22 , a signal (9.76 ppm) was found at lower field in comparison with that of [Ag 2 (dppb) 2 ] 2+ (−1.60 ppm) (dppb = 1,4-bis-(diphenylphosphino)butane). This fact indicates that certain intermediates containing phosphines were formed in the reaction, which are helpful for the protection of silver ions (Supplementary Fig. 1 ). We also obtained crude samples of Ag 21 with either Ph 3 P or dppm (bis(diphenylphosphino)methane) instead of dppb (Supplementary Fig. 2 ). In addition, the reduction process could be largely inhibited under basic conditions [37] . It was known that the species reduces gold(I) is BH 3 OH − , which comes from the hydrolysis of BH 4 − [38] . The hydrolysis was catalyzed by H + , so in basic solutions, the reduction process becomes more slowly [39] . A rapid reduction without MeONa gave a red solution that showed a broad plasmonic resonance absorption peak at ~450 nm, which indicates the formation of nanoparticles instead of clusters (Supplementary Fig. 3 ). Mass spectrometry and optical properties The positive ESI-MS spectrum of Ag 21 shows the molecular ion peak at m / z = 4307.71, corresponding to the monocation [Ag 21 (dpa) 12 ] + (calcd 4307.87) (Fig. 1a ), and the spectrum of Ag 22 gave signal of a dication [Ag 22 (dpa) 12 ] 2+ at m / z = 2207.39 (Fig. 1b ). The observed isotopic patterns of the clusters are both in perfect agreement with their simulated. X-ray photoelectron spectroscopy (XPS) revealed that the Ag3d 5/2 binding energy in Ag 21 and Ag 22 were observed at 368.0 and 368.2 eV, respectively, which suggested that the oxidation state of Ag were closer to Ag(0) (367.9 eV) (Supplementary Fig. 4 ). Fig. 1 ESI mass and optical absorption spectra of Ag 21 and Ag 22 in CH 2 Cl 2 . Mass spectra of Ag 21 ( a ) and Ag 22 ( b ), inset: the measured (black trace) and simulated (red trace) isotopic distribution patterns of the corresponding the molecular ion peaks. c UV-vis absorption spectra with photographs of Ag 21 (left) and Ag 22 (right) under ambient light. d Photon-energy plot in CH 2 Cl 2 Full size image In CH 2 Cl 2 , Ag 21 is a brown red solution, while Ag 22 is green. The UV/Vis spectrum of Ag 21 shows optical absorption bands at 352, 422, 520 and 576 nm (shoulder), whereas Ag 22 has absorptions at 354, 437, 505 and 582 nm (Fig. 1c ). In detail, the absorption peak in Ag 21 at 422 nm red shifts to 437 nm, while, the peak at 520 nm blue shifts to 505 nm in Ag 22 . Specifically, the first absorption peak at 576 nm in Ag 21 becomes more prominent in Ag 22 and red shifts to 582 nm. These spectral differences can also be observed in the photon-energy plots (Fig. 1d ). By extrapolating the absorbance to zero, the optical energy gaps were determined to be 1.92 eV for Ag 21 and 1.80 eV for Ag 22 , respectively. The difference in the optical properties of the two similar clusters indicates that the surface units have a significant disturbance to the electronic and optical properties [25] , [40] . Molecular structures Single crystal structural analysis revealed that Ag 21 comprises a monocation cluster [Ag 21 (dpa) 12 ] + while the Ag 22 cluster contains a dication cluster [Ag 22 (dpa) 12 ] 2+ of C 3 symmetry, both clusters have SbF 6 − counteranions. Both clusters consist of a centered-icosahedron Ag 13 core, and the surrounding protection are provided by 12 dpa ligands. The C 3 axis passes through the central Ag atom and the centers of two (opposite) triangular faces of Ag 12 icosahedron (Fig. 2a, b ). Eight Ag atoms caps the Ag 3 faces of the icosahedron in Ag 21 . Two of them lie on the C 3 axis and the remaining six locate around the C 3 axis in three groups alongside the icosahedron (Fig. 2c, d ). Thus, the ideal symmetry of the Ag 21 core is D 3h . Similarly, nine of the twenty Ag 3 faces of the icosahedron are capped by 9 Ag atoms to form a Ag 22 cluster and they are related by a C 3 axis (Fig. 2e ). Among them, three are located at the bottom, and the remaining six Ag atoms form three Ag 2 pairs (Fig. 2f ). In the Ag 13 core of Ag 21 , the center-surface Ag ⋯ Ag distances are in the range of 2.757–2.832 Å with an average value of 2.790 Å, while the surface–surface Ag ⋯ Ag distances are in the range of 2.770–3.168 Å with an average value of 2.933 Å. The values are comparable with the Ag···Ag distances of icosahedron Ag 13 observed in [Ag 35 (H 2 L) 2 (L)(C≡CBu t ) 16 ](SbF 6 ) 3 (H 4 L, p -tert-butylthiacalix[4]-arene) [41] (2.778 and 2.923 Å). Moreover, the distances of capping Ag atoms to Ag 13 kernel have an average value of 2.867 Å, while the average distances between capping atoms are 3.054 Å, indicating a compact contact between capping atoms to the Ag 13 kernel. 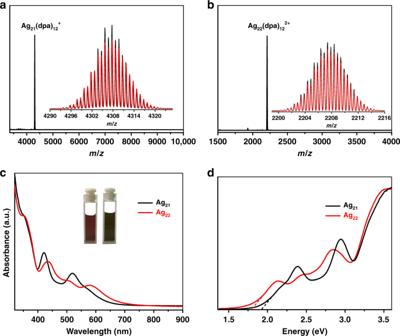Fig. 1 ESI mass and optical absorption spectra ofAg21andAg22in CH2Cl2. Mass spectra ofAg21(a) andAg22(b), inset: the measured (black trace) and simulated (red trace) isotopic distribution patterns of the corresponding the molecular ion peaks.cUV-vis absorption spectra with photographs ofAg21(left) andAg22(right) under ambient light.dPhoton-energy plot in CH2Cl2 Similar Ag ⋯ Ag bond distances were also observed in Ag 22 (Supplementary Table 1 ). Fig. 2 Molecular structures of Ag 21 and Ag 22 . Total structure of [Ag 21 (dpa) 12 ] + ( a ) and [Ag 22 (dpa) 12 ] 2+ ( b ) showing the Ag 13 polyhedron; Top view ( c ) and side view ( d ) of the Ag 21 kernel; Top view ( e ) and side view ( f ) of the Ag 22 kernel. Color codes: purple and green sphere, Ag; blue sphere, N; gray sphere, C Full size image The main structural feature in the two Ag clusters is that various interfacial binding geometries generated by dpa ligands. The dpa ligand has three coordination donors (one amido N donor and two pyridine N donors). It function as efficient surface protecting ligands, and there are four types of binding motifs of dpa with silver atoms presented in Ag 21 and Ag 22 (Fig. 3 ). In Ag 21 , three dpa ligands can be viewed as simple bridging groups (motif A) and six dpa ligands adopt μ 3 -bridging mode coordinating three silver atoms with each N donor ligating a Ag (motif B) (Supplementary Fig. 5 ). Only motif B has been previously found in Ag cluster [42] and the two binding modes have been also reported in other transition metals (e.g., Cr, Mo) [43] , [44] . Interestingly, the amido N of dpa could also ligate two metal atoms (motif C and motif D), so that the maximum coordination number of dpa can be 4. The two binding modes have never been reported before. The icosahedral Ag 12 cores of Ag 21 and Ag 22 are connected to three pyridine N atoms and nine amido N atoms (Supplementary Figs. 5 and 6 ). The 12 dpa ligands in Ag 22 adopt three different binding modes: six in motif B, three in motif C and three in motif D (Supplementary Fig. 6 ). The N py ⋯ Ag bond lengths in Ag 21 are in the range of 2.108–2.371 Å and the N amido ⋯ Ag bond lengths range from 2.042 to 2.510 Å. Similar values are also found in Ag 22 . (Supplementary Table 1 ). Fig. 3 Schematic representation of the binding modes of dpa in Ag 21 and Ag 22 Full size image The arrangements of the silver atoms and dpa ligands are shown in Fig. 4 . The conversion from Ag 21 to Ag 22 can be structurally understood as following: with the addition of a silver atom (bright green) to the surface of Ag 21 , the two cap silver atoms (yellow) move far apart from each other and the other two (dark green) twist their orientation significantly (Fig. 4a vs 4b ). The surface dpa ligands can be divided into four groups as marked in different color in Fig. 4c, d . The positions of dpa ligands are just slightly changed, which allows the addition one silver ion to the Ag 21 core or removal of one silver ion from the Ag 22 core. Detailed surface structural comparison is presented in Supplementary Fig. 7 . Fig. 4 Structural comparison of Ag 21 and Ag 22 . Kernel structures ( a vs b ) and surface ligand arrangements ( c vs d ) of [Ag 21 (dpa) 12 ] + and [Ag 22 (dpa) 12 ] 2+ Full size image Interconversion The flexible arrangement of the three N donors of dpa makes it possible to adjust the coordination positions of dpa, which is an important prerequisite for cluster interconversion. It was found that there is a solvent-dependent equilibrium between Ag 21 and Ag 22 (Fig. 5a ). The interconversion process can be monitored with absorption spectroscopy, because they have significantly different absorption profiles. The interconversion involves the adding or leaving of a Ag + ion on the surface structure of the clusters. The single Ag-species should hardly affect the absorption spectra due to its d [10] nature. As shown in Fig. 5b , Ag 22 dissolved in a mixture of EtOH and n-hexane (v: v = 1: 4) exhibits very similar profile to that of the freshly prepared Ag 21 . As the ratio of n-hexane to EtOH increases, the peak at 582 nm became weaker. Meanwhile, the peaks at 505 and 437 nm became stronger and they were shifted to 520 and 422 nm, respectively. These changes indicates that [Ag 22 (dpa) 12 ] 2+ has been gradually converted into [Ag 21 (dpa) 12 ] + . It is worth mentioning that three isosbestic points were observed at ~565, 500 and 435 nm in the UV-vis absorption spectra, which indicates one-to-one conversion stoichiometry from Ag 22 to Ag 21 . Moreover, the Ag 22 species could be recovered by increasing the ratio of EtOH to n-hexane (Supplementary Fig. 8 ). Both clusters have identical icosahedral Ag 13 cores, and the positions of their dpa ligands are just slightly changed. So, in the interconversion, the surface structure of the cluster only need to slightly adjust for the taking or releasing a Ag + ion. It should be mentioned that both Ag 21 and Ag 22 carry a valence electron count of 8e. The isoelectronic nature also contribute to the easy and reversible interconversion of these two nanoclusters. Fig. 5 The reversible interconversion between Ag 22 and Ag 21 . a Solvent-dependent equilibrium between Ag 21 and Ag 22 . Color codes: purple, green, and bright green sphere, Ag; blue sphere, N; gray sphere, C. b UV-vis spectra of Ag 22 dissolved in mixed solvents with various ratios of EtOH to n-hexane (the total volume of EtOH and n-hexane is kept the same). c UV-vis spectra of Ag 22 dissolved in a mixture of EtOH and n-hexane (v : v = 1 : 4) at different temperatures. ESI-MS spectra: d Ag 22 dissolved in EtOH. e Formation of Ag 21 cluster from Ag 22 when the volume ratio of EtOH to n-hexane is 1: 4. f Recovery of Ag 22 from Ag 21 when the volume ratio of EtOH and n-hexane is changed back to 9 : 1 Full size image The solvent-triggered interconversion was also confirmed by ESI-MS (Fig. 5d–f ). When the ratio of EtOH to n-hexane was 1: 4, Ag 21 species was detected as a prominent peak at m / z = 4307.80 ([Ag 21 (dpa) 12 ] + , Fig. 5e ), and the recovery of Ag 22 from Ag 21 was also verified by ESI-MS (Fig. 5f ). The prominent peak at m / z = 2207.26 was assigned to [Ag 22 (dpa) 12 ] 2+ , and the two small peaks with lower m/z values are [Ag 21 (dpa) 12 ] 2+ at 2153.76 (calcd 2153.93) and [Ag 20 (dpa) 12 ] 2+ at 2099.27 (calcd 2099.48), which are fragment ions after losing one or two Ag(0). The small peak at 2253.27 is [Ag 22 (dpa) 12 (EtOH) 2 ] 2+ (calcd 2253.43). Interestingly, the interconversion are also sensitive to temperature (Fig. 5c ). Lower temperature such as −20 °C favors the formation of Ag 22 species, and the reverse transformation to Ag 21 happened when the temperature of the solution was elevated to room temperature. Both Ag 21 and Ag 22 are soluble in ethanol, and the solubility of Ag 21 is 14 times as much as that of Ag 22 . As the arrangement of protecting ligands are very similar on the surface of both nanoclusters, the different solubility is largely due to that Ag 21 is +1 charged and Ag 22 carries two positive charges. Both clusters are not soluble in n-hexane, but Ag 21 is still soluble in the mixed solution of ethanol/n-hexane due to its excellent solubility in ethanol. As for Ag 22 , its solubility is significantly decreased as the increasing of the content of n-hexane in the mixed solution of ethanol/n-hexane, which forces the equilibrium moving to the formation of much more soluble Ag 21 . Control experiments were carried out to make sure that there is no concentration effect. The UV-vis spectra of EtOH solutions containing different concentration of Ag 21 or Ag 22 were measured. As shown in Supplementary Fig. 9 , the absorption peaks become weaker as the concentrations decrease, but no transformation occurred. Since the absorbance is proportional to the concentration of Ag 21 or Ag 22 , following the Lambert–Beer law, no aggregation occurs. Therefore, it is reasonable to conclude that the interconversion between Ag 22 and Ag 21 in solution is due to their largely different solubility. This statement is also supported by the temperature-dependent interconversion as above-mentioned (Fig. 5c ). Recently, Xie et al. revealed a size conversion reaction from [Au 23 ( p -MBA) 16 ] − to [Au 25 ( p -MBA) 18 ] − ( p -MBA = para-mercaptobenzoic acid), which could be induced by changing the solvent polarity (e.g., from water/ethanol to pure water) [45] . This work is certainly a different case. In summary, we have synthesized two all-amido-protected metal nanoclusters, and achieved their total structure determination. The flexible arrangement of the three N donors of dpa facilitates the formation of various interfacial Ag-N binding geometries, which favors the generation of cluster diversity. The solvent-triggered reversible interconversion presents an access for the atomic-level tailoring of the nanocluster structures and the regulation of their properties. The role of solvents on the transformation of cluster species and even nanoparticles is worth noting, which presents possibilities in obtaining desired clusters or particles in a convenient way. On the other hand, four binding modes of the dpa ligand have been revealed, and the coordination of dpa highlights its promising potential to act as a protecting agent in the formation of metal nanoclusters. This work sheds light on understanding of the metal−amido interface and the mechanism of the cluster conversion, which will stimulate the investigation on metal nanoclusters or even nanoparticles containing ligands of various amines. Chemicals and materials In all, 2, 2′-dipyridylamine, Sodium methanolate (MeONa, 98%) and Silver hexafluoroantimonate (AgSbF 6 , 98.0%) were purchased from J&K; sodium borohydride (NaBH 4 , 98%) and other reagents employed were purchased from Sinopharm Chemical Reagent Co. Ltd. (Shanghai, China). Other reagents employed were commercially available and used as received. Synthesis of dpaAg To a solution of AgNO 3 (500 mg, 2.94 mmol) in H 2 O (4 mL) and MeOH (100 mL), a solution of Hdpa (554 mg, 3.2 mmol) in MeOH (10 mL) was added under stirring. Then 612 µL of NEt 3 (446 mg, 4.46 mmol) was added to the solution, a light yellow precipitate was produced. The mixture was stirred for 30 min at room temperature in air in the dark. Then the solution was filtered to give a light yellow solid, which was washed with water (2 × 5 mL), ethanol (5 mL) and ether (5 mL) to give 728.6 mg (89% yield based on Ag) of dpaAg. Synthesis of Ag 21 (dpa) 12 (SbF 6 ) (Ag 21 ) To 2 mL CH 2 Cl 2 suspension containing dpaAg (27 mg, 0.1 mmol), dppb (8 mg, 0.019 mmol), and Hdpa (17 mg, 0.1 mmol), and 1 mL AgSbF 6 (5 mg) in MeOH and 1 mL 2 M MeONa (11 mg, 0.2 mmol) in MeOH were added. After stirring for 30 min, a freshly prepared solution of NaBH 4 (0.15 mg in 1.0 mL of ethanol) was added dropwise with vigorous stirring. The solution color changed from light yellow to reddish-brown, and the reaction continued overnight. Then the reaction was evaporated to dryness to give a reddish-brown solid. The solid was washed with n-hexane (2 × 3 mL), then dissolved in 3 mL CH 2 Cl 2 : toluene (v : v = 3 : 1), and the resulted solution was centrifuged for 3 min at 10,000 r.min −1 . The reddish-brown supernatant was collected and subjected to vapor diffusion with ether: n-hexane (v : v = 1: 5) to afford reddish-brown crystals after 7 days in 5.2 mg yield (24% based on Ag). Anal. UV-vis (λ, nm): 352; 422; 520; 576 (shoulder peak). 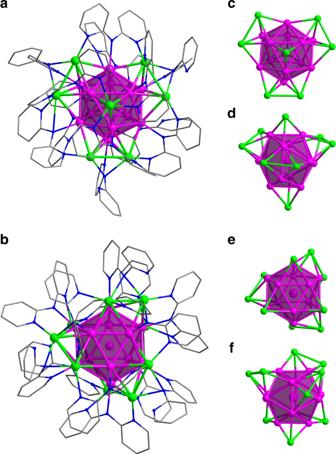Fig. 2 Molecular structures ofAg21andAg22. Total structure of [Ag21(dpa)12]+(a) and [Ag22(dpa)12]2+(b) showing the Ag13polyhedron; Top view (c) and side view (d) of the Ag21kernel; Top view (e) and side view (f) of the Ag22kernel. Color codes: purple and green sphere, Ag; blue sphere, N; gray sphere, C (E, eV): 3.54; 2.94; 2.39; 2.17. Eg = 1.92 eV. ESI-MS (CH 2 Cl 2 ): 4307.71 ([Ag 21 (dpa) 12 )] + ). XPS (binding energy, eV): Ag 3d 5/2 , 368.0; Ag 3d 3/2 , 374.0 eV. Synthesis of Ag 22 (dpa) 12 (SbF 6 ) 2 (Ag 22 ) To 2 mL CH 2 Cl 2 suspension containing dpaAg (27 mg, 0.1 mmol) and dppb (8 mg, 0.019 mmol), 1 mL AgSbF 6 (5 mg) in MeOH and 1 mL 2 M MeONa (11 mg, 0.2 mmol) in MeOH were added. After stirring for 30 min, a freshly prepared solution of NaBH 4 (0.10 mg in 1.0 mL of ethanol) was added dropwise with vigorous stirring. The solution color changed from light yellow to green, and the reaction continued overnight. Then the reaction was evaporated to dryness to give a green solid. The solid was washed with ether: n-hexane (v : v = 1 : 3) (5 mL), then dissolved in 3 mL CH 2 Cl 2 : toluene (v : v = 3 : 1), and the resulted solution was centrifuged for 3 min at 10,000 r.min −1 . The green supernatant was collected and subjected to vapor diffusion with ether: n-hexane (v : v = 1 : 5) to afford black crystals after 10 days in 5 mg yield (20% based on Ag). Anal. UV-vis (λ, nm): 354; 437; 505; 582. (E, eV): 3.52; 2.85; 2.44; 2.13. Eg = 1.80 eV. ESI-MS (CH 2 Cl 2 ): 2207.41 ([Ag 22 (dpa) 12 )] 2+ ). XPS (binding energy, eV): Ag 3d 5/2 , 368.2; Ag 3d 3/2 , 374.2 eV. General procedure for transformation 20 mg Ag 22 was dissolved in 1 mL EtOH, and the solution was divided into 10 portions of 30 μL. Then, different volume of EtOH and n-hexane were added, and make sure the total volume is 3 mL. With the increase of the ratio of n-hexane, the color of the solution gradually changed from green to red. For the reverse transformation, different volume of EtOH and n-hexane were added to the obtained red solution in the same method. With the increase of the ratio of EtOH, the red solution gradually return back to green. The transformation was very fast, which was monitored by measuring UV-Vis absorption spectra of the mixture after gentle shaking. Physical measurements UV-Vis absorption spectra was recorded on a Shimadzu UV-2550 Spectrophotometer. Mass spectrum was recorded on an Agilent Technologies ESI-TOF-MS. Fourier-transform infrared spectroscopy (FT-IR) spectra were collected in the range of 4000–400 cm −1 with a Bruker FT-IR spectrometer. Nuclear magnetic resonance (NMR) data were collected on a JEOL ECS-400 spectrometer. X-ray photoelectron spectroscopy (XPS) studies were performed on PHI Quantum-2000 XPS. The sample was put under UHV to reach the10 −8 Pa range. The non-monochromatized Al Kα source was used at 10 kV and 10 mA. All binding energies were calibrated using the C (1s) carbon peak (284.6 eV), which was applied as an internal standard. High resolution narrow-scan spectra were recorded with the electron pass energy of 50 eV and takeoff angle of 55° to achieve the maximum spectral resolution. X-ray crystallography Intensity data of Ag 21 and Ag 22 were collected on an Agilent SuperNova Dual system (Cu Kα) at 180 K and 173 K, respectively. 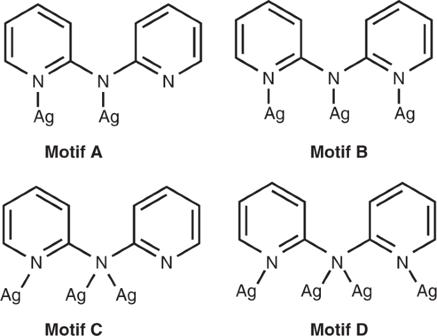Fig. 3 Schematic representation of the binding modes of dpa inAg21andAg22 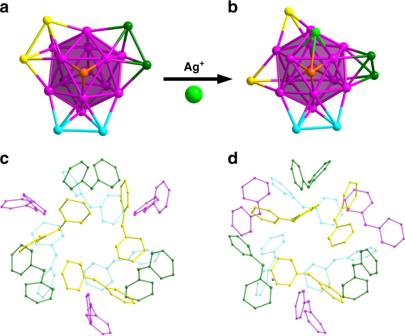Fig. 4 Structural comparison ofAg21andAg22. Kernel structures (avsb) and surface ligand arrangements (cvsd) of [Ag21(dpa)12]+and [Ag22(dpa)12]2+ 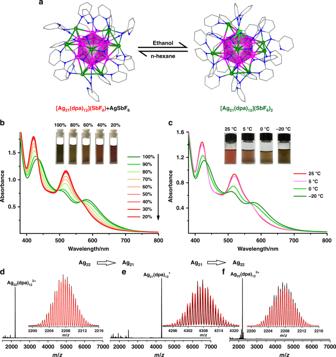Fig. 5 The reversible interconversion betweenAg22andAg21.aSolvent-dependent equilibrium betweenAg21andAg22. Color codes: purple, green, and bright green sphere, Ag; blue sphere, N; gray sphere, C.bUV-vis spectra ofAg22dissolved in mixed solvents with various ratios of EtOH to n-hexane (the total volume of EtOH and n-hexane is kept the same).cUV-vis spectra ofAg22dissolved in a mixture of EtOH and n-hexane (v : v = 1 : 4) at different temperatures. ESI-MS spectra:dAg22dissolved in EtOH.eFormation ofAg21cluster fromAg22when the volume ratio of EtOH to n-hexane is 1: 4.fRecovery ofAg22fromAg21when the volume ratio of EtOH and n-hexane is changed back to 9 : 1 Absorption corrections were applied by using the program CrysAlis (multi-scan) and all the structures were solved by direct methods. All non-hydrogen atoms of Ag 22 were refined anisotropically by least-squares on F 2 using the SHELXTL program. The hydrogen atoms of organic ligands were generated geometrically. Ag atoms of Ag 21 were refined with anisotropic displacement parameters, while others were refined with isotropic atomic displacement parameters. SQUEEZE routine in PLATON was employed in the structural refinements.